Structure and compatibility of a magnesium electrolyte with a sulphur cathode Magnesium metal is an ideal rechargeable battery anode material because of its high volumetric energy density, high negative reduction potential and natural abundance. Coupling Mg with high capacity, low-cost cathode materials such as electrophilic sulphur is only possible with a non-nucleophilic electrolyte. Here we show how the crystallization of the electrochemically active species formed from the reaction between hexamethyldisilazide magnesium chloride and aluminum trichloride enables the synthesis of a non-nucleophilic electrolyte. Furthermore, crystallization was essential in the identification of the electroactive species, [Mg 2 (μ-Cl) 3 ·6THF] + , and vital to improvements in the voltage stability and coulombic efficiency of the electrolyte. X-ray photoelectron spectroscopy analysis of the sulphur electrode confirmed that the electrochemical conversion between sulphur and magnesium sulfide can be successfully performed using this electrolyte. Energy diversification is necessary for global sustainability and the minimization of industrial and automotive pollution. Low-cost, high energy density batteries utilizing environmentally friendly elements used for storing intermittent energy from renewable resources such as solar and wind are bound to increase in demand. High energy density, rechargeable batteries will have a large role in powering market-competitive electric vehicles, where the available space to mount the battery packs dictates the volumetric energy density is more important than gravimetric energy density. Attractive choices are alkaline/alkaline earth metal anodes, which provide some of the highest theoretical volumetric capacities of any anode material: the volumetric capacity of lithium, sodium, calcium and magnesium are 2,062, 1,128, 2,073 and 3,832 mAh cm −3 , respectively. For comparison, current graphite anodes for lithium-ion batteries have a volumetric capacity of 777 mAh cm −3 . Additionally, metallic anodes do not require solid-state diffusion of ions to transfer material from the charged to the discharged state, but merely the successful deposition/dissolution of the ions onto/from the surface of the metal. Magnesium metal has a high negative reduction potential (−2.356 V versus NHE) and the highest volumetric capacity of the practical choices from group I and II metals (beryllium metal is not a practical choice because of its high cost of $7,480 per kg), which make it a superior alternative as an anode material for high energy density batteries [1] . Furthermore, Mg is not plagued by dendrite formation, which is a significant safety issue that has dissuaded the commercialization of rechargeable batteries utilizing a lithium metal anode [2] , [3] , [4] . The first rechargeable batteries with Mg metal anodes were demonstrated in 2000. These Mg batteries showed impressive cycle life (>3,500 cycle measured), low capacity fading over prolonged cycling, negligible self-discharge and wide temperature operating range [5] . However, these batteries were then considered only as replacements for nickel–cadmium or lead–acid batteries because the high formula weight of the Chevrel phase Mg x Mo 3 S 4 cathode lowered the overall energy density. Further research on alternative high-energy Mg battery systems has also been hindered by the surface chemistries of Mg, which greatly limits the choice of available electrolytes and cathodes [6] , [7] . With regard to high-energy systems, one of the ideal materials to couple Mg with is sulphur [8] , which has a high theoretical capacity (1,671 mAh g −1 or 3,459 mAh cm −3 ). The combination of a magnesium anode and a sulphur cathode is of great interest because the theoretical energy density of this battery is estimated to be over 4,000 Wh l −1 , which is approximately twice that of a Li ion battery composed of a graphite anode and a cobalt oxide cathode. Unfortunately, Mg electrolytes reported so far [6] , [9] , [10] , while having high coulombic efficiencies, are nucleophilic, and, therefore, preclude the use of electrophilic cathodes such as sulphur. Consequently, the feasibility and performance of a Mg/S battery is completely unknown, because there is no electrolyte compatible with both Mg and S. To couple the two electrodes, an electrolyte able to transport Mg 2+ ions between the anode and cathode is essential. In general, the prerequisites for battery electrolytes include electrochemical/chemical stability, ionic conduction and electronic insulation [4] . Magnesium organohaloaluminate electrolytes, generated in situ from the reaction between a Lewis acid and a Lewis base, are nucleophilic. For example, a 2:1 mixture of phenylmagnesium chloride and aluminum trichloride (AlCl 3 ) in tetrahydrofuran (THF) is incompatible with an electrophilic sulphur cathode. Gas chromatography–mass spectroscopy analysis confirmed that this electrolyte directly reacts with sulphur to form phenyl disulphide and biphenyl sulphide. Consequently, our synthetic strategy was to avoid a direct reaction with sulphur by focusing on utilizing non-nucleophilic bases. The fact that potassium hexamethyldisilazide (KN(SiMe 3 ) 2 ) is a non-nucleophilic base suggests that hexamethyldisilazide magnesium chloride (HMDSMgCl) is an excellent candidate, because it has been reported to be capable of reversible Mg deposition [10] . Unfortunately, the coulombic efficiency, voltage stability and current density of the HMDSMgCl electrolyte are far inferior to magnesium organohaloaluminate electrolytes, and, as a result, it has not received much attention. Here we report the performance enhancement of HMDSMgCl, through the addition of a Lewis acid AlCl 3 . Crystallization of the electrochemically active species resulted in a dramatic improvement in the potential stability and coulombic efficiency and, furthermore, it is the critical step in synthesizing a non-nucleophilic electrolyte that is chemically compatible with an electrophilic sulphur cathode. Although the dissolution of sulphur and polysulphides plagues the Mg/S system with rapid fade, we demonstrate a proof of concept for the first rechargeable Mg/S battery. Electrochemical analysis of the electrolyte To enhance the electrochemical performance of the HMDSMgCl electrolyte, we investigated its reactivity with a Lewis acid, AlCl 3 . By varying the ratio of acid to base and the reaction time, we found the optimum electrochemical performance of the electrolyte to be when the ratio of HMDSMgCl:AlCl 3 was 3:1 and the reaction time was 24 h. It is noteworthy to state that organomagnesium chemistry is acutely sensitive to moisture and air, and, therefore, all reactions and electrochemical experiments were performed in a glovebox under an argon atmosphere. 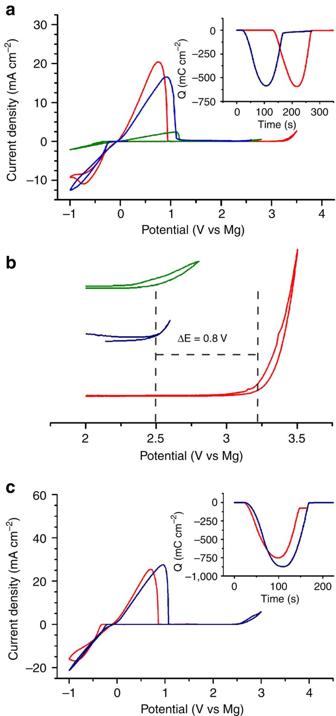Figure 1: Electrochemical performance of Mg electrolytes. (a) Cyclic voltammograms of HMDSMgCl (green), the reaction product generatedin situfrom a 3:1 mixture of HMDSMgCl to AlCl3(blue), and the crystal obtained from a 3:1 mixture of HMDSMgCl to AlCl3(red). Inset shows the charge balance during the deposition and the subsequent dissolution of Mg. (b) Enlargement of 2–3.5 V region of (a)highlighting the oxidative stability of the electrolytes. (c) Cyclic voltammograms of 0.4 M THF solution of the reaction product generatedin situfrom a 2:1 mixture of Bu2Mg to EtAlCl2(blue), and the crystal obtained from a 2:1 mixture of Bu2Mg to EtAlCl2(red). Scan rate for all cyclic voltammograms are 0.025 V s−1. The current density for Mg deposition is increased by almost a factor of seven by the addition of AlCl 3 , as shown by the green and blue lines in Figure 1a . Unfortunately, the voltage stability of the HMDSMgCl electrolyte was not improved ( Fig. 1b ). To clarify the product from the reaction between HMDSMgCl and AlCl 3 , a crystal was obtained by slow diffusion of hexane. The crystal structure [Mg 2 (μ-Cl) 3 ·6THF][HMDSAlCl 3 ], 1 , was determined by single-crystal X-ray diffraction ( Fig. 2 ), which was solved to reveal a cation consisting of two octahedrally coordinated Mg centres bridged by three chlorine atoms. The three remaining sites on each Mg are occupied by THF molecules coordinated through the oxygen. The counter anion is an aluminum atom tetrahedrally coordinated by one HMDS group and three chlorine atoms. The [Mg 2 (μ-Cl) 3 ·6THF] + cation has been previously isolated in the solid state from a THF-based Grignard reagent solution [11] , from the selective synthesis of a 1,3,4-triphospholide anion [12] , and from a catalytic metathesis reaction between ZnCl 2 and t BuMgCl (ref. 13 ). Figure 1a compares the electrochemical activity of the crystal redissolved in THF (red) to that of the electrolyte generated in situ from the reaction between HMDSMgCl and AlCl 3 (blue). It is impressive that the voltage stability of the electrolyte increased by almost 0.8 V after crystallization. We propose that the purification step removes any unreacted HMDSMgCl, that starts to electrochemically oxidize and decompose around 2.5 V. This is supported by spiking the redissolved, crystallized electrolyte with a HMDSMgCl solution, which results in a decrease of voltage stability from 3.2 to 2.5 V. In addition, crystallization of the electrolyte increases the coulombic efficiency from 95 to 100%, as shown in Figure 1a , inset. The superior electrochemical performance of the crystal 1 , is fascinating, considering its structural similarity to the allegedly inactive crystal, [Mg 2 (μ-Cl) 3 ·6THF][C 2 H 5 AlCl 3 ]. This crystal was reported to be obtained from an active electrolyte composed of di-n-butylmagnesium ([CH 3 (CH 2 ) 3 ] 2 Mg, Bu 2 Mg) and ethylaluminum dichloride (C 2 H 5 AlCl 2 , EtAlCl 2 ), but electrochemically inactive when dissolved in THF [5] . This contradiction prompted us to reevaluate the electrochemical performance of the crystals obtained from the reaction product of Bu 2 Mg and EtAlCl 2 . We found the crystal was indeed electrochemically active, although the coulombic efficiency was reduced from 100 to 90% ( Fig. 1c , and inset). Figure 1: Electrochemical performance of Mg electrolytes. ( a ) Cyclic voltammograms of HMDSMgCl (green), the reaction product generated in situ from a 3:1 mixture of HMDSMgCl to AlCl 3 (blue), and the crystal obtained from a 3:1 mixture of HMDSMgCl to AlCl 3 (red). Inset shows the charge balance during the deposition and the subsequent dissolution of Mg. ( b ) Enlargement of 2–3.5 V region of ( a) highlighting the oxidative stability of the electrolytes. ( c ) Cyclic voltammograms of 0.4 M THF solution of the reaction product generated in situ from a 2:1 mixture of Bu 2 Mg to EtAlCl 2 (blue), and the crystal obtained from a 2:1 mixture of Bu 2 Mg to EtAlCl 2 (red). Scan rate for all cyclic voltammograms are 0.025 V s −1 . 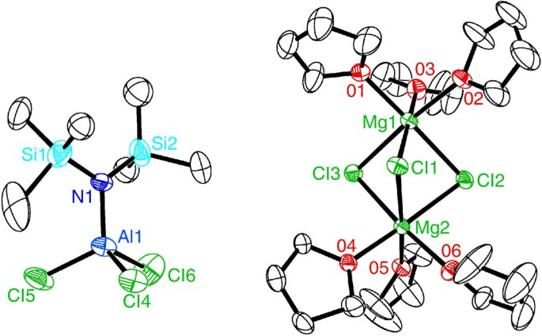Figure 2: Structure of the crystallized product, 1. ORTEP plot (25% thermal probability ellipsoids) of [Mg2Cl3-6THF][HMDSAlCl3]. Hydrogen atoms, THF of crystallization and second component of disorder are omitted for clarity. Full size image Figure 2: Structure of the crystallized product, 1. ORTEP plot (25% thermal probability ellipsoids) of [Mg 2 Cl 3 -6THF][HMDSAlCl 3 ]. Hydrogen atoms, THF of crystallization and second component of disorder are omitted for clarity. Full size image Chemical analysis of the electrolyte The 1 H NMR spectrum of the white crystalline product obtained from the reaction mixture of HMDSMgCl and AlCl 3 (3:1) dissolved in d 8 -THF displayed 2 singlets at 0.12 and −0.01 p.p.m.. The 13 C {1H} NMR spectrum shows 3 resonances, two high frequency peaks assigned to the protic THF atoms and the peak at 6.1 p.p.m. assigned to the -CH 3 groups of the HMDS ligand. The 27 Al and the 25 Mg NMR both displayed a broad singlet peak at 103.9 and 5.02 p.p.m., respectively. The mass spectroscopy analysis showed an exact mass and isotope pattern consistent with both an HMDSAlCl 3 − anion and an HMDS 2 AlCl 2 − anion. Based on the fact that the HMDSAlCl 3 − anion will be shifted further downfield than the HMDS 2 AlCl 2 − anion, we assign the peak at 0.12 p.p.m. to the methyl protons of 1 , and the peak at −0.01 p.p.m. to the same group in [Mg 2 (μ-Cl) 3 ·6THF][HMDS 2 AlCl 2 ], 1 . The integration of the two peaks clearly shows that the ratio of 1 to 1 is 97:3. Unfortunately, we could not observe the [HMDS 2 AlCl 2 ] − co-product by 13 C NMR owing to the low yield. However, we feel the presence is sufficiently evidenced through mass spectroscopy and 1 H NMR analysis. Equations (1,2,3,4) show the proposed key step in the formation of 1 as the transmetallation of the HMDS group to yield the HMDSAlCl 3 − anion [equation (1)]. The resulting MgCl + cation is not observed, and one plausible scenario to account for the cation in 1 is that the MgCl + rapidly reacts with MgCl 2 [equation (3)]. Some MgCl 2 is present from the Schlenk equilibrium [equation (2)], and depletion of the MgCl 2 drives the equilibrium to the right. Evidence for the formation of HMDS 2 Mg was confirmed through 1 H NMR by spiking the original reaction mixture with a commercial sample of HMDS 2 Mg. A proposed pathway to account for the minor product, 1 , involves the reaction of 1 with HMDSMgCl [equation (5)]. Evidence for this reaction was found by increasing the concentration of HMDSMgCl and the reaction time, which consequently amplified the percentage of 1 formed. As affirmation of the compatibility, we investigated the reactivity of the electrolyte with elemental sulphur through NMR. We observed no change in the 33 S NMR of elemental sulphur in the presence of the electrolyte, even after one week. The 1 H, 13 C and 27 Al NMR of the electrolyte also remains unchanged in the presence of elemental sulphur. Based on the NMR studies, the non-reactive nature of the electrolyte with sulphur clearly demonstrates that the electrolyte is indeed non-nucleophilic and therefore chemically compatible with an electrophilic sulphur cathode. X-ray photoelectron spectroscopy of the sulphur cathode Our non-nucleophilic electrolyte is the key that opens the door to examining the performance of a Mg/S battery. Coin cells with a metallic magnesium anode, separator, and a sulphur cathode consisted of elemental sulphur dispersed in carbon black and a polymeric binder, were assembled to test the feasibility of our electrolyte. 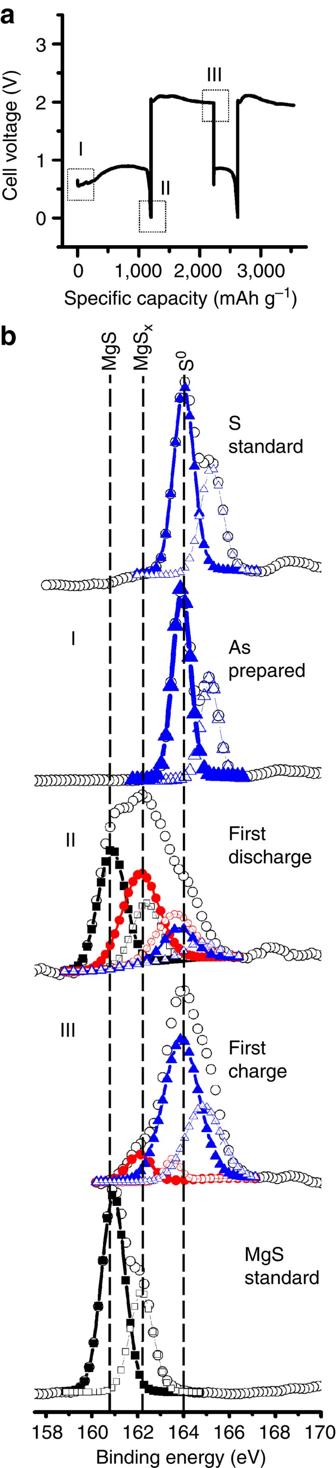Figure 3: XPS analysis of sulphur cathode. (a) Discharge and charge of a Mg/S coin cell at 50 and 25 μA, respectively. XPS spectra were taken from coin cells at various stages of cycling. (b) HRES S 2p spectra of the cathode as-prepared (I), after first discharge (II) and after first charge (III) are compared with standard samples of S powder (top) and MgS powder (bottom). Note that the S 2p peaks contain both a 2p3/2and 2p1/2spin-orbit splitting state. The 2p3/2states, located at lower binding energies, were used for chemical state identification and are emphasized with filled symbols. As Figure 3a shows, a typical Mg/S coin cell displayed an excellent capacity of 1,200 mAh g −1 (2,484 mAh cm −3 , based on the mass of sulphur) for the first discharge. The starting potential is 0.55 V and slowly increases up to 0.89 V during the discharge process. The rise is most likely due to the fracturing of the resistive surface layer on the magnesium anode, evidenced by the higher voltage at the start of the second discharge, when the surface layer is no longer present. The second discharge capacity dramatically decreased to 394 mAh g −1 (816 mAh cm −3 ), which stimulated our investigations into the reasons for the large capacity fade. Figure 3: XPS analysis of sulphur cathode. ( a ) Discharge and charge of a Mg/S coin cell at 50 and 25 μA, respectively. XPS spectra were taken from coin cells at various stages of cycling. ( b ) HRES S 2p spectra of the cathode as-prepared (I), after first discharge (II) and after first charge (III) are compared with standard samples of S powder (top) and MgS powder (bottom). Note that the S 2p peaks contain both a 2p 3/2 and 2p 1/2 spin-orbit splitting state. The 2p 3/2 states, located at lower binding energies, were used for chemical state identification and are emphasized with filled symbols. Full size image To examine the components after undergoing a discharge/charge cycle, we dismantled a Mg/S coin cell for visual inspection and chemical analysis. The apparent yellow discolouration of the separator indicated that the main cause of capacity fade is polysulphide or sulphur dissolution [14] , which also explains the overcharging behaviour observed in Figure 3a . We note that our preliminary coin cells are not optimized to prevent sulphide dissolution, and therefore display typical problems of a S cathode. Polysulphide dissolution, a rapid capacity fade, and overcharging are well-known problems in Li/S battery system [15] . Polysulphides can be charged to various chain lengths and migrate between the anode and cathode via a sulphide shuttle mechanism. During overcharge of Li/S battery, soluble polysulphides are formed on the cathode, diffuse to the anode to be reduced there, and, then, diffuse back to the cathode to be reoxidized. Consequently, the current can continue to flow without actually oxidizing Li 2 S to S, or 'recharging' the battery. One of the most direct ways to gain a deeper understanding of the battery chemistry is X-ray photoelectron spectroscopy (XPS), because it can determine the change in the oxidation state of sulphur on the surface of the cathode as the result of battery cycling. Figure 3b compares high-resolution (HRES) S 2p spectra obtained from sulphur cathodes (as-prepared, after a first discharge, and after a complete discharge/charge cycle), to standard samples of S and magnesium sulphide (MgS) powder. The as-prepared sulphur cathode was composed of elemental sulphur and is evidenced by the S 2p 3/2 peak located at 164.0 eV. After discharging the Mg/S coin-cell, the oxidation state of the sulphur in the cathode changed dramatically. Curve-fit analysis of the S 2p peak showed that three oxidation states of sulphur were present. As expected from the battery chemistry, the majority of the sulphur was reduced to lower oxidation states indicated by the lower binding energies. The 2p 3/2 peak positioned at 160.9 eV confirmed the conversion to MgS. The extra peaks observed between S and MgS are most reasonably assigned to magnesium polysulphides (MgS x , 1<×<8, S 2p 3/2 =162.0–163.0 eV), because a non-stoichiometric presence of magnesium cations will shift the S 2p peaks to slightly lower binding energies than sulphur, but slightly higher binding energies than the fully reduced MgS. Our rationale for the peak positions of polysulphides is consistent with XPS HRES spectra of cleaved NiS surfaces [16] . Furthermore, our analysis is in accordance with the multiple peaks observed at higher binding energies than LiS in the S 2p spectra of lithium stored in polysulphide solutions [17] . After re-charging, the majority of sulphur returns to S 0 , with a small contribution from MgS x , which confirms the successful transition between S and MgS via a polysulphide intermediate. Several mechanisms for the deposition of Mg from active electrolytes are presented in literature. Various analytical approaches, such as in situ Fourier transform infrared spectroscopy, single crystal X-ray diffraction, Raman spectroscopy, multinuclear NMR, and X-ray absorption fine structure have been used to elucidate the structure of the electrochemically active species in magnesium organohaloaluminate electrolytes [5] , [7] , [18] , [19] , [20] , [21] . Several conclusions have been drawn. The active species in the solution comprises MgCl + and Mg 2 Cl 3 + cations and AlR 4−n Cl n ( n =1–3) anions; THF molecules are also incorporated in the chemical structure of the active species, and [Mg 2 (μ-Cl) 3 ·6THF][C 2 H 5 AlCl 3 ] solid product, obtained from an active electrolyte solution composed of Bu 2 Mg and EtAlCl 2 , is electrochemically inactive when dissolved in THF. Attempts to understand the mechanism for the deposition of Mg have been hamstrung by the inability to isolate an electrochemically active species from the magnesium organohaloaluminate electrolytes. Here we contradict previous findings where [Mg 2 (μ-Cl) 3 ·6THF][C 2 H 5 AlCl 3 ], obtained from an active electrolyte composed of di-n-butylmagnesium and ethylaluminum dichloride, is electrochemically inactive when dissolved in THF [5] . We found that the structurally analogous [Mg 2 (μ-Cl) 3 ·6THF][HMDSAlCl 3 ] crystal is electrochemically active when obtained from the reaction of HMDSMgCl and AlCl 3 . This suggests that the [Mg 2 (μ-Cl) 3 ·6THF] + cation present in both electrolytes, is the electroactive species generated by the reaction between an organomagnesium compound and a Lewis acid. However, we cannot discard the fact that the [Mg 2 (μ-Cl) 3 ·6THF] + cation may be in equilibrium with MgCl 2 and MgCl + ; hence, we cannot be confident that the [Mg 2 (μ-Cl) 3 ·6THF] + cation is entirely responsible for Mg deposition. Future work to understand the deposition mechanism, including in situ electrochemical/X-ray absorption fine structure analysis, will shed light on the exact role of the active [Mg 2 (μ-Cl) 3 ·6THF] + cation during Mg deposition/dissolution. The unique chemical reactions of individual battery electrodes present new challenges to developing the next generation of high-energy density batteries. Nucleophilic, organomagnesium compounds are, ironically, pivotal in synthetic organic chemistry, but detrimental to electrophilic cathodes such as sulphur. By crystallizing the electrochemically active species from a 3:1 mixture of HMDSMgCl:AlCl 3 , we mitigated the nucleophilic attack on the sulphur cathode. The increased coulombic efficiency and wider voltage window were electrochemical benefits also achieved through crystallization. XPS analysis provided us a method to monitor the electrochemical conversion of the cathode as it was charged and discharged. A yellow discolouration of the separator, during a visual inspection of a dismantled coin cell, and subsequent XPS analysis of the cathode, revealed that the sulphur cathode still suffered from similar challenges as Li/S batteries do. In addition, when compared with Li systems, Mg is substantially plagued by polysulfide and sulphur dissolution due to the THF solvent that is a crucial component of the electrochemically active species [Mg 2 (μ-Cl) 3 ·6THF] + . Unfortunately, other common battery solvents such as carbonates are reduced on Mg metal and form a passivating solid electrolyte interface that prevents Mg deposition. A possible reason to explain the discharge capacity being greater than the charge capacity is polysulfide migration between the anode and cathode by a shuttling mechanism. The major advantage of magnesium metal is the lack of dendrite formation at the anode surface that is a major capacity and safety issue that hinders Li metal systems. Research on Li/S batteries suggests that one of the most promising approaches to improving the performance of the sulphur cathode is S–C nanocomposites [22] . Furthermore, a key challenge in developing a Mg/S battery is the discovery of new solvents with low solubility of polysulfides and sulphur that are not reduced on the magnesium anode. In summary, we report the performance enhancement of HMDSMgCl through the addition of a Lewis acid AlCl 3 . Here we characterize the electrochemically active species [Mg 2 (μ-Cl) 3 ·6THF] + formed from the reaction of an Hauser base compound HMDSMgCl and a Lewis acid AlCl 3 . This crystallization resulted in a dramatic improvement in the potential stability and coulombic efficiency, and, furthermore, it is the critical step in synthesizing a non-nucleophilic electrolyte that is chemically compatible with an electrophilic sulphur cathode. AlCl 3 in THF In an argon-filled glovebox, a 250 ml Schlenk flask is outfitted with a powder addition funnel and stir bar. The flask is charged with 60 ml anhydrous THF and cooled to 0 °C. AlCl3 (5.0 g, 37.5 mmol, 99.999%, Sigma-Aldrich) is added via the powder addition funnel, at a rate to avoid an exothermic reaction. This reaction was allowed to slowly warm to room temperature once all the AlCl 3 was added. A clear solution resulted, which was diluted to 75 ml total volume. HMDSMgCl in THF A 250 ml 3-neck flask is outfitted with a nitrogen inlet/outlet, stir bar, reflux condenser, addition funnel, and a heating mantle. The apparatus is flushed with nitrogen and charged with 50 ml anhydrous THF and freshly distilled hexamethyldisilazane (23.8 g, 147 mmol, >99.0%, Fluka). Freshly prepared ethyl magnesium chloride (EtMgCl, 70 ml, 140 mmol in THF) is added slowly via the addition funnel and the mixture is refluxed until the EtMgCl is completely consumed, as indicated by phenanthroline. The reaction is refluxed for 8 h. Once all EtMgCl is consumed extra EtMgCl is added in 0.5 ml portions with refluxing until an excess persists. This excess EtMgCl is then carefully back-titrated in a similar manner with further hexamethyldisilazane until the end point is achieved. The final concentration is determined by titration with diphenylacetic acid. Preparation of (Mg 2 (μ-Cl) 3 ·6THF)(HMDS n AlCl 4−n ) ( n =1, 2) In an argon-filled glovebox, AlCl 3 (0.5 M solution in THF, 3 ml, 1.5 mmol) was mixed with 3 equivalents of freshly prepared HMDSMgCl (1.44 M solution in THF, 3.125 ml, 4.5 mmol) in a 20 ml screw capped vial. The vial was immediately capped and vigorously stirred for 24 h. The crystals were formed by slow diffusion of anhydrous hexane (Sigma-Aldrich, 6 ml). The resulting crystals were washed with hexane and dried under vacuum to furnish ~800 mg of white crystalline product. (60% yield) 1 H-NMR (d 8 -THF, 500 MHz): δ 0.12 p.p.m. (s, CH 3 groups on 1 ), −0.01 (s, CH 3 groups on 1 ). 13 C-NMR (d 8 -THF, 500 MHz): δ 68.4, 26.4, 6.1. 27 Al-NMR (d 8 -THF, 500 MHz): δ 103.9. 25 Mg-NMR (d 8 -THF, 300 MHz): δ 5.00. Crystallography Crystal data for C 34 H 74 AlCl 6 Mg 2 NO 7 Si 2 ; M r =953.42; Monoclinic; space group P2 1 /c; a =11.6517(7) Å; b =13.6722(8) Å; c =32.490(2) Å; α =90°; β =93.9030(10)°; γ =90°; V =5163.8(5) Å 3 ; Z =4; T =200(2) K; λ (Mo-K α )=0.71073 Å; μ (Mo-K α )=0.459 mm −1 ; d calc =1.226g cm −3 ; 52,464 reflections collected; 8,792 unique ( R int =0.0386); giving R 1 =0.0846, w R 2 =0.2347 for 5610 data with [ I >2 σ ( I )] and R 1 =0.1228, w R 2 =0.2713 for all 8,792 data. Residual electron density (e − .Å −3 ) max/min: 1.245/−0.493. An arbitrary sphere of data were collected on a colourless rod-like crystal, having approximate dimensions of 0.50 mm×0.27 mm×0.20 mm, on a Bruker Kappa X8-APEX-II diffractometer using a combination of ω- and ϕ-scans of 0.5° (ref. 23 ). Data were corrected for absorption and polarization effects and analysed for space group determination [24] . The structure was solved by direct methods and expanded routinely. The model was refined by full-matrix least-squares analysis of F 2 against all reflections. All non-hydrogen atoms were refined with anisotropic thermal displacement parameters. Unless otherwise noted, hydrogen atoms were included in calculated positions. Thermal parameters for the hydrogens were tied to the isotropic thermal parameter of the atom to which they are bonded (1.5× for methyl, 1.2× for all others). Methyl groups on the ((Me) 3 Si) 2 AlNCl 3 anion were found to be disordered. The methyl carbon positions were located at the ellipse locii that described the elongated thermal envelope. These half-occupancy carbon atoms were then refined with isotropic thermal parameters. Large thermal motion, bordering on disorder, was also observed in all THF moieties. It was decided that refinement, as an anisotropic model, led to an overall satisfactory structure. The disorder results in a lower-than-desired maximum angle for observed data as well as unusual thermal parameter relationships. Carbon atoms in the THF and methyl groups typically have thermal parameter envelopes greater than their neighbouring atoms, whereas the heavier atoms are more well-located and have smaller thermal displacement ellipsoids than their neighbouring carbon atoms. This pseudo-disorder results in a larger number of alerts, beyond those immediately addressed. However, the conclusions drawn by the structure are not affected by the thermal motion of peripheral atoms. Hydrogen atoms were all included in geometrically calculated positions. Electrochemistry All solutions were diluted to 0.4 M with regard to Mg. Cyclic voltammograms were obtained using a Solartron 1,287 potentiostat in a conventional 3-electrode cell with a Pt disk working electrode, a Mg wire reference electrode, and a Mg ribbon counter electrode at a scan rate of 0.025 V s −1 . All Measurements were performed in an argon-filled glovebox. Battery Coin cells were built in an argon-filled glovebox using standard parts for 2032-type cells. Anodes comprised 100-μm-thick Mg foil (ESPI Metals). Cathodes were prepared by coating sulphur–carbon composite ink (61% elemental sulphur, 35% carbon black, 4% poly(tetrafluoroethylene) binder) on a porous carbon substrate. Cathode analysis The XPS analyses were carried out with a PHI5802 Multitechnique instrument using a monochromatic Al Kα source (1486.6 eV). Air-sensitive samples were transferred into the instrument under inert gas environments. Non-linear least squares curve-fitting was applied to selected HRES spectra ( χ 2 <1). NMR spectroscopy All NMR experiments were performed at magnetic field strengths of 11.7 ( 1 H, 13 C, 27 Al) and 7.05 ( 25 Mg, 33 S) T corresponding to 1 H resonance frequencies of 499.89 and 299.89 MHz, respectively, and at ambient temperature (~21 °C) using Varian Inova and UnityPlus spectrometers. The Varian Inova spectrometer was equipped with a 5 mm broadband probe to measure one-dimensional (1D) 1 H, 13 C, and 27 Al spectra. The Varian UnityPlus spectrometer was equipped with a 10 mm broadband probe to measure 1D 25 Mg and 33 S spectra. Usually 20 mg of sample were dissolved in 0.6 ml of THF-d 8 . Chemical shift values δ are given in p.p.m.. 1 H and 13 C spectra were referenced to residual solvent signals; δ =1.73 for 1 H and δ =25.4 for 13 C. 25 Mg, 27 Al, and 33 S spectra were referenced indirectly using external reference standards ( δ =0) MgCl 2 , Al(NO 3 ) 3 , and saturated ammonium sulphate, respectively, in D 2 O. How to cite this article: Kim, H. S. et al . Structure and compatibility of a magnesium electrolyte with a sulphur cathode. Nat. Commun. 2:427 doi: 10.1038/ncomms1435 (2011).